Crossreactivity of a human autoimmune TCR is dominated by a single TCR loop Self-reactive CD4 T cells are thought to have a central role in the pathogenesis of many chronic inflammatory human diseases. Microbial peptides can activate self-reactive T cells, but the structural basis for such crossreactivity is not well understood. The Hy.1B11 T cell receptor (TCR) originates from a patient with multiple sclerosis and recognizes the self-antigen myelin basic protein. Here we report the structural mechanism of TCR crossreactivity with two distinct peptides from human pathogens. The structures show that a single TCR residue (CDR3α F95) makes the majority of contacts with the self-peptide and both microbial peptides (66.7–80.6%) due to a highly tilted TCR-binding topology on the peptide-MHC surface. Further, a neighbouring residue located on the same TCR loop (CDR3α E98) forms an energetically critical interaction with the MHC molecule. These data show how binding by a self-reactive TCR favors crossreactivity between self and microbial antigens. Autoimmune diseases such as multiple sclerosis (MS), type 1 diabetes and rheumatoid arthritis have a complex pathogenesis. Genome-wide studies have identified large numbers of genes that contribute to disease susceptibility and epidemiological studies have implicated environmental factors [1] , [2] . Infectious agents may contribute to the pathogenesis of autoimmune diseases by inducing the activation and clonal expansion of self-reactive lymphocytes [3] . A large body of work showed that self-reactive human and murine T cells can be activated by microbial peptides that meet the structural requirements for MHC binding and T cell receptor (TCR) recognition, and studies in experimental animal models demonstrated that TCR crossreactivity can induce an autoimmune process [4] , [5] , [6] , [7] , [8] . Activation of self-reactive T cells by microbial peptides with sufficient sequence similarity has also been referred to as ‘molecular mimicry’ [9] , [10] . It was initially thought that such crossreactivity would be a rare event, but a large number of studies have shown that it is an inherent property of TCR recognition [11] . Experiments with combinatorial peptide libraries demonstrated that a substantial number of stimulatory peptides could be identified for individual T cell clones [5] . In fact, important aspects of T cell biology require TCR activation by crossreactive peptides: positive selection of T cells in the thymus is induced by MHC-bound self-peptides, and these peptides are usually unrelated to microbial peptides recognized by these T cells later in their lifespan [12] . Furthermore, survival of naive T cells in peripheral lymphoid organs requires continuous exposure to endogenous peptides [13] , [14] . Crossreactivity has been invoked to explain recognition of virtually any MHC-bound peptide by the TCR repertoire present in an individual. It has also been shown to be beneficial in the settings of chronic infection by rapidly mutating pathogens because it increases the probability that pathogen-specific T cells retain reactivity to mutated microbial epitopes [15] . Crossreactivity also accounts for the high frequency of alloreactive T cells following organ transplantation [15] . In several cases, TCR crossreactivity was explained by substantial flexibility of TCR CDR3 loops, which are located at the centre of the TCR interface with peptide/MHC (pMHC) [16] , [17] . This conclusion is supported by the observation that the CDR3 loops can have different conformations in free and pMHC-bound states [18] , [19] , [20] . Flexibility of the peptide, and less frequently of the MHC molecule, can also contribute to TCR crossreactivity [17] . Crossreactivity can also result from entirely different TCR-binding interactions between self- and allo-pMHC ligands, as shown first for the 2C TCR [21] , [22] . The distinct binding interface of 2C TCR with the allo-ligand (H-2 L d -QL9) was due to substantial rotation of the TCR on the pMHC surface compared with the self-ligand (H-2 K b -dEV8) [21] . Structural studies on both murine and human self-reactive TCRs have identified features of pMHC binding that can differ from the majority of anti-microbial TCRs. Two general categories of self-reactive TCRs can be distinguished based on the eight structures that have been determined: (1) TCR-binding topologies that differ substantially from those observed for anti-microbial TCRs. Such binding topologies can also affect the geometry of CD4 engagement and may thereby impact early signalling events during T cell development [23] , [24] , [25] , [26] ; (2) TCRs that bind self-pMHC in a canonical diagonal orientation but engage self-ligands with structural defects or suboptimal MHC anchors [23] , [24] , [27] , [28] , [29] , [30] , [31] , [32] , [33] . It is thought that destabilization of self-reactive TCR-pMHC complexes by one of these two mechanisms contributes to escape from negative selection by self-reactive T cells in the thymus. Little is still known about the structural mechanisms of TCR crossreactivity in autoimmune diseases, and only one structure had been determined. The Ob.1A12 TCR was isolated from a patient with relapsing–remitting MS and recognized a myelin basic protein (MBP) peptide bound to HLA-DR15 (ref. 34 ). This TCR showed a binding topology to HLA-DR15/MBP that differed significantly from most anti-microbial TCRs: the TCR was shifted towards the peptide N terminus and also rotated counter-clockwise relative to the axis of the bound peptide [23] . This TCR crossreacted with a bacterial engA peptide when it was processed from a complete antigen, and injection of this bacterial peptide aggravated CNS inflammation in a HLA-DR15/Ob.1A12 TCR transgenic mouse model [35] . The structure with the HLA-DR15/engA peptide also showed a shift towards the peptide N terminus, and the CDR3 loops interacted in a similar manner with HLA-DR15-bound MBP and bacterial engA peptides [35] . However, there were substantial differences in the conformation of the germline-encoded CDR2α and CDR2β loops as well as a 3° rotation of the TCR between the two structures [23] , [35] . The Hy.1B11 TCR originated from a patient with relapsing–remitting MS and was specific for a peptide from MBP (res. 85–99) bound to HLA-DQ1 (DQ1; DQA1 *0102, DQB1 *0502) [27] , [34] . We previously showed that the human Hy.1B11 T cell clone was not only activated by MBP but also by four peptides from human pathogens that were quite distinct from MBP and each other [4] . Previous studies also provided evidence for in vivo expansion of T cells expressing the Hy.1B11 TCR: the same α and β chain sequences were isolated from three independent clones (originating from two different blood samples drawn 13 months apart) [36] . Such in vivo expansion may have been caused by recognition of a crossreactive antigen or MBP. The structure of Hy.1B11 TCR bound to DQ1/MBP peptide revealed a binding mode in which the TCR was strongly tilted relative to the DQ1/peptide surface. As a consequence, the germline-encoded loops of the TCRα chain (CDR1α and CDR2α) did not bind to DQ1, and the peptide was contacted by only one of the CDR3 loops (CDR3α but not CDR3β). In this study, we define the structural basis for crossreactivity between the MBP self-peptide and two peptides from human pathogens for Hy.1B11 TCR. These DQ1/microbial peptide complexes are recognized by Hy.1B11 TCR with the same highly tilted binding mode as the DQ1/MBP peptide complex. These results are explained by the dominant contribution of a single TCR residue, CDR3α F95, to recognition of both self and microbial peptides. Structure determination We determined the crystal structures of the trimolecular TCR–pMHC complex for two microbial peptides that activated Hy.1B11 T cells. These peptides originated from the UL15 terminase protein of Herpes simplex virus (UL15 154–166 , abbreviated as UL15) and the phosphomannomutase protein of Pseudomonas aeruginosa (PMM 260–274 , abbreviated as PMM). The structures were determined to a resolution of 2.2 Å (UL15 peptide) and 2.86 Å (PMM peptide) ( Supplementary Table S1 ). Both complexes had one molecule in the asymmetric unit with very similar unit cell dimensions to each other and the Hy.1B11–DQ1/MBP complex. Further, both structures showed excellent electron density at the interface of TCR, peptide and DQ1 ( Supplementary Fig. S1 ). There was poor density for DQα 44–52 in the trimolecular complex with the MBP peptide, but this segment had a helical conformation in the structures with UL15 and PMM peptides (this part of the molecule forms a short 3 10 helix in most HLA class II molecules and interacts with HLA-DM) [37] . The UL15 and PMM peptides were quite diverse in their sequence from the MBP peptide and each other ( Fig. 1 ). Each of the microbial peptides shared three residues with the MBP peptide, which included P3 Phe (both UL15 and PMM), P1 Val and P2 His (UL15) as well as P5 Lys and P8 Val (PMM). The position of the conserved P3 Phe within the DQ1 binding groove was very similar among the three trimolecular complexes ( Fig. 1a,b ). This result was consistent with previous mutagenesis data that identified P3 Phe as a key TCR contact residue of the MBP peptide: among 18 tested single amino-acid analogues of the MBP peptide, only three had activity (P3 Tyr, Met and Gly, albeit at significantly lower levels) [27] . The MBP, PMM and UL15 peptides also shared a positive charge at P5 (Lys in MBP and PMM, Arg in UL15) ( Fig. 1c ). Outside this core region, the three peptides differed substantially in their sequence as well as the conformation of particular segments. For example, the MBP and PMM peptides showed notable differences in the conformation of the N-terminal (P1–P3) peptide segment ( Fig. 1a ). 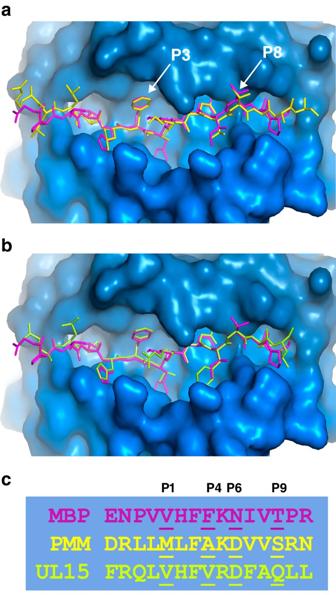Figure 1: Comparison of DQ1-bound self and microbial peptides. (a,b) Conformation of microbial peptides in the DQ1 binding site. PMM (yellow,a) and UL15 (green,b) peptides are compared with MBP peptide (magenta;a,b). DQ1 is shown as a surface and the three peptides as stick models; Hy.1B11 TCR has been omitted for clarity. Peptide positions P3 and P8 are indicated (a). (c) Alignment of PMM and UL15 peptides with MBP self peptide. DQ1 anchor residues (P1, P4, P6 and P9) are indicated. Figure 1: Comparison of DQ1-bound self and microbial peptides. ( a , b ) Conformation of microbial peptides in the DQ1 binding site. PMM (yellow, a ) and UL15 (green, b ) peptides are compared with MBP peptide (magenta; a , b ). DQ1 is shown as a surface and the three peptides as stick models; Hy.1B11 TCR has been omitted for clarity. Peptide positions P3 and P8 are indicated ( a ). ( c ) Alignment of PMM and UL15 peptides with MBP self peptide. DQ1 anchor residues (P1, P4, P6 and P9) are indicated. Full size image TCR contacts with DQ1-bound peptides The interaction of Hy.1B11 TCR with MBP and microbial peptides was characterized by a striking feature, the deep insertion of the CDR3α F95 side chain into a pocket created by the P2, P3 and P5 peptide residues ( Fig. 2a–c ). The surface area of CDR3α F95 that became solvent inaccessible was similar among the three complexes, 163.6 Å 2 (MBP), 154.5 Å 2 (PMM) and 171.4 Å 2 (UL15). This TCR side chain formed the majority of peptide contacts in all three complexes, ranging from 66.7–80.6% of all TCR-peptide contacts in the three structures ( Table 1 ). CDR3α F95 formed a close stacking interaction with the P3 Phe peptide residue, and the carbonyl oxygen of the CDR3α F95 backbone formed a hydrogen bond with P5 Lys/Arg of MBP, PMM and UL15 peptides. CDR3α E98 also interacted with P5 Lys/Arg of the three complexes but measured distances were outside the range of optimal hydrogen bond formation (3.5–3.8 Å) except in the case of P5 Lys in PMM where the distance was 3.2 Å ( Fig. 2 ). 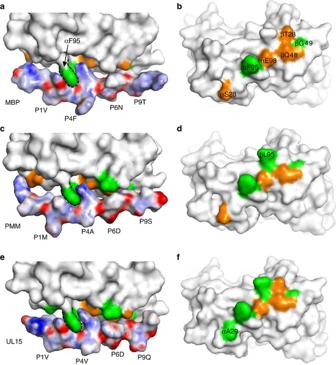Figure 2: Deep insertion of TCR CDR3α F95 into a pocket created by three peptide residues. (a–c) Interaction of Hy.1B11 TCR with MBP, PMM and UL15 peptides. TCR and peptides are rendered as surfaces, whereas DQ1 has been omitted to improve peptide visualization, MBP (a) PMM (b) and UL15 (c). TCR residues that contact peptides are coloured based on their biochemical properties (hydrophobic—green, polar—orange). Peptide residues are coloured based on charge (acidic—red, basic—blue). Peptide anchor residues (P1, P4, P6 and P9) as well as TCR CDR3α F95 are indicated. (d–f) TCR contact surface for MBP, PMM and UL15 peptides. View is rotated by 90° relative toa–c, and TCR residues contacting MBP (d) PMM (e) and UL15 (f) peptides are indicated. Figure 2: Deep insertion of TCR CDR3α F95 into a pocket created by three peptide residues. ( a – c ) Interaction of Hy.1B11 TCR with MBP, PMM and UL15 peptides. TCR and peptides are rendered as surfaces, whereas DQ1 has been omitted to improve peptide visualization, MBP ( a ) PMM ( b ) and UL15 ( c ). TCR residues that contact peptides are coloured based on their biochemical properties (hydrophobic—green, polar—orange). Peptide residues are coloured based on charge (acidic—red, basic—blue). Peptide anchor residues (P1, P4, P6 and P9) as well as TCR CDR3α F95 are indicated. ( d – f ) TCR contact surface for MBP, PMM and UL15 peptides. View is rotated by 90° relative to a – c , and TCR residues contacting MBP ( d ) PMM ( e ) and UL15 ( f ) peptides are indicated. Full size image Table 1 Peptide contacts by Hy.1B11 TCR. Full size table Further analysis of the critical CDR3α F95 residue showed π–π stacking interactions involving three residues, with P2 His being positioned between CDR3α F95 and DQ1β H81 ( Fig. 3 ). This stacking interaction was very similar among complexes involving MBP or UL15 peptides, which shared a histidine residue at P2. The PMM peptide carried a leucine residue at P2, which disrupted the π–π stacking arrangement and increased the overall distance between CDR3α F95 and DQ1β H81 by 1.5 Å. Loss of the stacking arrangement also reduced the number of interactions between CDR3α F95 and P2 (15 in MBP versus 5 in PMM). Movement of CDR3α F95 away from P2 Leu of the PMM peptide brought it closer to the hydrophobic part of the P5 Lys side chain with which it made more extensive contacts compared to the structure with the MBP peptide. In the structure with the UL15 peptide, a sulphate ion was coordinated by P5 Arg of the peptide and two other arginine residues (TCRα R51 and DQ1β R77), but surface plasmon resonance experiments showed that addition of sulphate did not enhance Hy.1B11 TCR binding in the presence of physiological NaCl concentrations ( Supplementary Fig. S2 ). 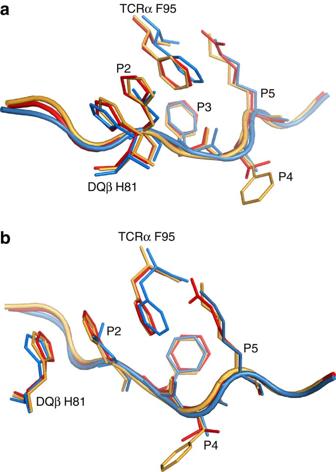Figure 3: Stacking interactions by peptide P2 histidine and TCR CDR3α F95. (a,b) Aromatic stacking interactions formed by CDR3α F95. P2 His forms π–π stacking interactions with DQ1 β81 His and TCR CDR3α F95 (residues from MBP structure in orange, UL15 in red and PMM in blue). P2 Leu in PMM peptide disrupts this π–π interaction, thereby affecting the position of both DQ1 β81 His and TCR CDR3α F95. TCR CDR3α F95 forms stacking interactions with P2 His (MBP, UL15) and P3 Phe (all peptides); in addition, it forms hydrophobic interactions with the P5 side chain (Lys/Arg). View inafrom peptide N terminus, inbfrom peptide C terminus. Figure 3: Stacking interactions by peptide P2 histidine and TCR CDR3α F95. ( a , b ) Aromatic stacking interactions formed by CDR3α F95. P2 His forms π–π stacking interactions with DQ1 β81 His and TCR CDR3α F95 (residues from MBP structure in orange, UL15 in red and PMM in blue). P2 Leu in PMM peptide disrupts this π–π interaction, thereby affecting the position of both DQ1 β81 His and TCR CDR3α F95. TCR CDR3α F95 forms stacking interactions with P2 His (MBP, UL15) and P3 Phe (all peptides); in addition, it forms hydrophobic interactions with the P5 side chain (Lys/Arg). View in a from peptide N terminus, in b from peptide C terminus. Full size image Outside of the P2–P5 core region, differences in Hy.1B11 TCR interaction with the three peptides were observed ( Figs 2 and 4 ). For example, the TCR interacted with different peptide positions and/or residues of the N-terminal peptide segment: P-3 Asn of MBP (with CDR1α S28), P-3 Arg of PMM (with CDR1α S28) and P-1 Leu of UL15 (with CDR1α A29) ( Table 1 ). Further, Hy.1B11 TCR interacted with the P7 peptide position in only two of the complexes and the actual peptide residues were different (P7 Val of PMM, P7 Phe of UL15) ( Fig. 4 , Table 1 ). The TCR contacted the P8 position of all three peptides, but all of these interactions appeared to be quite weak (see below), and there was variable involvement of TCR CDR1β T28 (MBP and UL15 peptides, but not PMM) ( Fig. 4 ). These results demonstrated the central role of CDR3α 95F in crossreactivity between self and microbial peptides by Hy.1B11 TCR. Outside of this core region, fewer TCR–peptide contacts were made, which were also more diverse among the three structures. 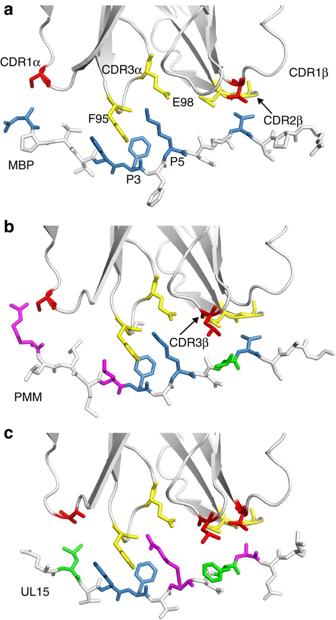Figure 4: Conserved and divergent features of Hy.1B11 TCR interaction with self and microbial peptides. (a–c) Interaction of TCR CDR loops with MBP and microbial peptides. CDR loops that contact MBP (a), PMM (b) and UL15 (c) peptides are shown. TCR residues forming similar contacts with all three peptides are coloured yellow, whereas TCR residues that make different contacts are highlighted in red. Peptide residues are coloured as follows: blue, sequence identity between microbial peptide and MBP; magenta, absence of sequence identity with MBP; green, TCR contact to PMM/UL15 peptides but not MBP peptide. Figure 4: Conserved and divergent features of Hy.1B11 TCR interaction with self and microbial peptides. ( a – c ) Interaction of TCR CDR loops with MBP and microbial peptides. CDR loops that contact MBP ( a ), PMM ( b ) and UL15 ( c ) peptides are shown. TCR residues forming similar contacts with all three peptides are coloured yellow, whereas TCR residues that make different contacts are highlighted in red. Peptide residues are coloured as follows: blue, sequence identity between microbial peptide and MBP; magenta, absence of sequence identity with MBP; green, TCR contact to PMM/UL15 peptides but not MBP peptide. Full size image TCR-binding topology The overall topology of Hy.1B11 TCR binding to the three DQ1–peptide complexes was very similar, as shown by pairwise superposition of trimolecular complexes with microbial peptides to the structure with the MBP peptide ( Fig. 5 ). The pairwise root-mean-square deviation for Cα residues was 0.53 for the trimolecular complexes with PMM and MBP peptides, and 0.48 for complexes with UL15 and MBP peptides. Thus, the Hy.1B11 TCR showed a highly tilted binding mode to all three DQ1/peptide complexes, which limited TCR interaction with the DQβ1 helix. The CDR loops of the TCR showed similar conformations, with little differences in their position; the largest change was a 1 Å movement of the tip of CDR3α in the PMM trimolecular complex compared with the two other structures. As a consequence, Hy.1B11 TCR formed a similar set of contacts with DQ1 in the three structures ( Supplementary Tables S2 and S3 ). 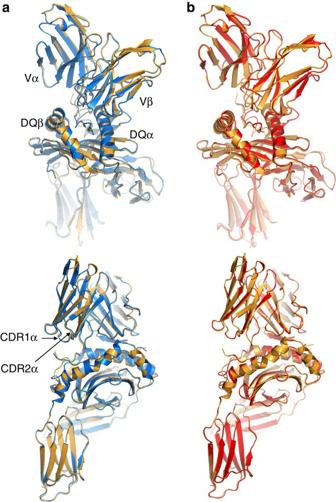Figure 5: Similar docking mode of Hy.1B11 TCR on self and microbial peptide/DQ1 complexes. (a,b) Tilted binding mode of Hy.1B11 TCR with DQ1/peptide complexes. Comparison of three crystal structures in which Hy.1B11 TCR recognizes distinct DQ1-bound peptides: MBP self-peptide (orange) as well as microbial peptides PMM (blue) and UL15 (red). Complexes were superimposed using the DQα chain to reveal any differences in TCR positioning. TCR, peptide and MHC are rendered as ribbon diagrams; TCR constant domains have been omitted for clarity. The trimolecular complexes are viewed from the peptide C terminus (top panels) and the DQ β1 helix (90° rotation, bottom panels). TCR Vα and Vβ domains, DQα and DQβ chains as well as TCR CDR1α and CDR2α loops are indicated. Figure 5: Similar docking mode of Hy.1B11 TCR on self and microbial peptide/DQ1 complexes. ( a , b ) Tilted binding mode of Hy.1B11 TCR with DQ1/peptide complexes. Comparison of three crystal structures in which Hy.1B11 TCR recognizes distinct DQ1-bound peptides: MBP self-peptide (orange) as well as microbial peptides PMM (blue) and UL15 (red). Complexes were superimposed using the DQα chain to reveal any differences in TCR positioning. TCR, peptide and MHC are rendered as ribbon diagrams; TCR constant domains have been omitted for clarity. The trimolecular complexes are viewed from the peptide C terminus (top panels) and the DQ β1 helix (90° rotation, bottom panels). TCR Vα and Vβ domains, DQα and DQβ chains as well as TCR CDR1α and CDR2α loops are indicated. Full size image We previously performed alanine-scanning mutagenesis of TCR residues that contacted the DQ1/MBP peptide surface and found that two mutations—CDR3α F95A and E98A—greatly reduced binding to DQ1/MBP ( K d >250 μM) [27] . SPR experiments showed that these two TCR residues were also critical for Hy.1B11 TCR binding to DQ1/UL15 and DQ1/PMM complexes ( Fig. 6c–f ). The impact of the CDR3α E98A mutation was particularly severe and little residual binding to DQ1 with bound PMM or UL15 peptides was detected even at high TCR concentrations. CDR3α E98 was part of a complex hydrogen bonding network, and it formed a salt bridge with DQ1α R61 as well as a hydrogen bond with CDR1β Y30 ( Fig. 6g and h ). These data demonstrated that F95A and E98A of CDR3α represented energetic ‘hotspots’ for peptide and DQ1 binding, respectively. 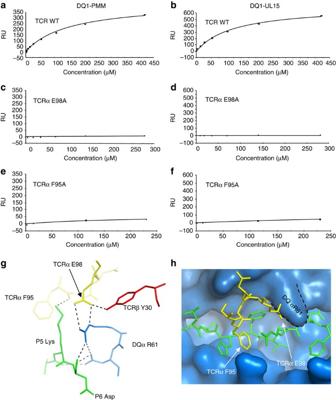Figure 6: Two residues at the tip of the CDR3α loop are critical for TCR binding to microbial peptides and DQ1. (a–f) Binding of TCR mutants to microbial DQ1/peptide complexes. Binding of Hy.1B11 WT and mutant TCRs (αE98A and αF95A) to DQ1/peptide was examined by surface plasmon resonance, as indicated on each graph. DQ1 proteins were mono-biotinylated on a BirA site located at the DQα C terminus and captured on streptavidin chips (1,500 RU). WT and mutant TCRs were injected over a range of concentrations (2 min at 25 °C, 15 μl min−1) into flow cells with immobilized DQ1/CLIP (negative control), DQ1/UL15 and DQ1/PMM. The signal from the DQ1/CLIP control flow cell was subtracted from experimental readings. Equilibrium binding constantKdwas calculated for binding of Hy.1B11 WT TCR to DQ1/PMM (a) and DQ1/UL15 (b) complexes using nonlinear curve fitting. Binding studies were performed at least twice with similar results. (g) Hydrogen bonding network formed by TCR CDR3α E98 with DQα R61 and CDR3 Y30. TCR loops are coloured yellow for CDR3α and red for CDR3β; the DQα chain is coloured blue and the PMM peptide green. (h) Interaction of the CDR3α loop (yellow) with the UL15 peptide (green) and DQ1 (blue, space-filling model). The DQ1α R61 residue forms a salt bridge with CDR3α E98. Figure 6: Two residues at the tip of the CDR3α loop are critical for TCR binding to microbial peptides and DQ1. ( a – f ) Binding of TCR mutants to microbial DQ1/peptide complexes. Binding of Hy.1B11 WT and mutant TCRs (αE98A and αF95A) to DQ1/peptide was examined by surface plasmon resonance, as indicated on each graph. DQ1 proteins were mono-biotinylated on a BirA site located at the DQα C terminus and captured on streptavidin chips (1,500 RU). WT and mutant TCRs were injected over a range of concentrations (2 min at 25 °C, 15 μl min −1 ) into flow cells with immobilized DQ1/CLIP (negative control), DQ1/UL15 and DQ1/PMM. The signal from the DQ1/CLIP control flow cell was subtracted from experimental readings. Equilibrium binding constant K d was calculated for binding of Hy.1B11 WT TCR to DQ1/PMM ( a ) and DQ1/UL15 ( b ) complexes using nonlinear curve fitting. Binding studies were performed at least twice with similar results. ( g ) Hydrogen bonding network formed by TCR CDR3α E98 with DQα R61 and CDR3 Y30. TCR loops are coloured yellow for CDR3α and red for CDR3β; the DQα chain is coloured blue and the PMM peptide green. ( h ) Interaction of the CDR3α loop (yellow) with the UL15 peptide (green) and DQ1 (blue, space-filling model). The DQ1α R61 residue forms a salt bridge with CDR3α E98. Full size image These experiments also showed that the binding affinity of the Hy.1B11 TCR was higher for DQ1/MBP (14.3±1.5 μM) than DQ1/PMM (154±18 μM) and DQ1/UL15 (124±5 μM) (all measurements at room temperature). The binding affinities of Hy.1B11 TCR for all three DQ1–peptide complexes were higher at 37 °C: 6.96±0.9 μM (DQ1/MBP), 57.3±1.6 μM (DQ1/PMM) and 51.6±2 μM (DQ1/UL15). ( Figs 6a and b and Supplementary Fig. S3 ), but they followed a similar trend consistent with previous data showing that the MBP peptide stimulated Hy.1B11 T cells at lower concentrations than PMM or UL15 peptides [4] . Nevertheless, the reduced TCR affinity was partially compensated by an increased binding affinity of PMM and UL15 peptides for DQ1, compared with the MBP peptide ( Fig. 7a ). We investigated the structural basis for the lower TCR-binding affinity to DQ1/UL15 and found that it could be largely attributed to the arginine at P5 (lysine in MBP): single amino-acid substitution from P5 Arg to Lys increased the affinity of the DQ1/UL15 complex to 23.8±2.2 μM ( Supplementary Fig. S4 ). This result was explained by steric hindrance due to the larger size of the guanidinium group, which resulted in suboptimal geometry for formation of an ideal hydrogen bond between the main chain carbonyl of CDR3α F95 and the guanidinium group of P5 Arg [38] . 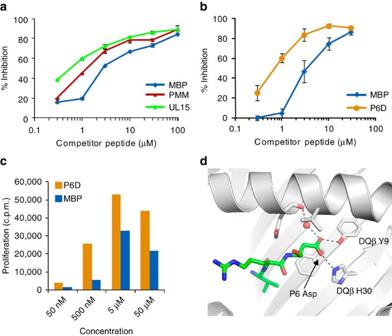Figure 7: Aspartic acid at P6 anchor position enhances DQ1 binding by microbial peptides. (a) UL15 and PMM peptides bind with higher affinity to DQ1 than the MBP peptide. Unlabelled MBP, UL15 or PMM peptides (0.3, 1, 3, 10, 30 and 100 μM) were used as competitors for DQ1 binding by a biotinylated MBP peptide (400 nM). Following overnight incubation at RT, DQ1/peptide complexes were captured by an immobilized antibody (9.3.F10), and DQ1-bound biotinylated peptide was detected using europium-labeled streptavidin. Data are shown as±s.d. Experiment was repeated three times with similar results (b) Competition binding assay performed as in (a) demonstrating enhanced DQ1 binding by MBP peptide with P6 Asn to Asp substitution. Data are shown as ±s.d. The experiment was carried out two times with similar results. (c) Enhanced proliferation of Hy.1B11 T cell clone to MBP P6 Asp analogue (orange) compared with MBP peptide (blue). (d) Interaction of P6 Asp with the P6 pocket of DQ1. Shown is the interaction of the UL15 peptide P6 side Asp side chain with DQβ H30 and DQβ Y9. DQ1 is shown as a cartoon and the peptide (P4-P6 segment) as a stick model. Figure 7: Aspartic acid at P6 anchor position enhances DQ1 binding by microbial peptides. ( a ) UL15 and PMM peptides bind with higher affinity to DQ1 than the MBP peptide. Unlabelled MBP, UL15 or PMM peptides (0.3, 1, 3, 10, 30 and 100 μM) were used as competitors for DQ1 binding by a biotinylated MBP peptide (400 nM). Following overnight incubation at RT, DQ1/peptide complexes were captured by an immobilized antibody (9.3.F10), and DQ1-bound biotinylated peptide was detected using europium-labeled streptavidin. Data are shown as±s.d. Experiment was repeated three times with similar results ( b ) Competition binding assay performed as in (a) demonstrating enhanced DQ1 binding by MBP peptide with P6 Asn to Asp substitution. Data are shown as ±s.d. The experiment was carried out two times with similar results. ( c ) Enhanced proliferation of Hy.1B11 T cell clone to MBP P6 Asp analogue (orange) compared with MBP peptide (blue). ( d ) Interaction of P6 Asp with the P6 pocket of DQ1. Shown is the interaction of the UL15 peptide P6 side Asp side chain with DQβ H30 and DQβ Y9. DQ1 is shown as a cartoon and the peptide (P4-P6 segment) as a stick model. Full size image Selection of an anchor residue that enhanced DQ1 binding The peptide residues occupying DQ1-binding pockets were considerably more diverse than the principal TCR contact residues. For example, all four anchor residues of the PMM peptide (P1, P4, P6 and P9) were distinct from the MBP peptide ( Figs 1 and 2 ). Nevertheless, the general biochemical properties of these DQ1 contacts showed similarities among the three peptides: the P1 and P4 anchor residues had a different degree of hydrophobicity, whereas the P6 and P9 anchor residues had polar side chains. Peptide-binding studies confirmed the degenerate binding specificities of the P4, P6 and P9 pockets ( Supplementary Table S4 ). The P4 pocket favored large hydrophobic anchor residues, whereas the P6 pocket showed a preference for small and acidic amino acids. In contrast, the P9 pocket could accommodate most side chains, and only large aromatic residues interfered with peptide binding. The UL15 and PMM peptides bound with higher affinity to DQ1 than the MBP peptide ( Fig. 7a ). This was surprising because the PMM peptide had a suboptimal anchor at the P4 position (alanine; phenylalanine in MBP peptide). The higher DQ1 affinity of both microbial peptides thus suggested a compensation mechanism. The four microbial peptides that stimulated the Hy.1B11 T cell clone shared an interesting feature: an aspartic acid at P6 (asparagine in MBP peptide) [4] . Peptide competition experiments demonstrated that a P6 Asn to Asp analogue peptide had a 10-fold higher affinity for DQ1 compared with the WT MBP peptide ( Fig. 7b , Supplementary Table S4 ). The functional relevance of P6 Asp was confirmed in T cell assays: a MBP P6 Asp analogue induced substantially stronger T cell proliferation compared with the MBP peptide, in particular at low peptide concentrations ( Fig. 7c ). Asparagine and aspartic acid are isosteric, and both can serve as hydrogen donors and acceptors; however, Asp can also participate in salt bridge formation. The P6 residue interacted with histidine and tyrosine residues in the P6 pocket (DQβ H30 and DQβ Y9) ( Fig. 7d ). In the microbial peptides, P6 Asp can form a buried salt bridge with this histidine, which would be energetically more favourable (~2 kcal mol −1 ) than the hydrogen bond formed by P6 Asn of MBP [39] . These results demonstrated the importance of P6 aspartic acid for DQ1 binding by the four microbial peptides. These data show that the Hy.1B11 TCR recognizes two distinct peptides from human pathogens with the same tilted binding topology as the human MBP peptide. In all three cases, two TCR residues formed critical interactions with the peptide (CDR3α F95) and DQ1 (CDR3α E98), respectively. These TCR residues were located within a four-residue segment at the tip of the CDR3α loop, and mutation of either residue to alanine greatly diminished binding to self and microbial peptide/DQ1 complexes. Particularly striking was the finding that a single residue (CDR3α F95) formed the majority of TCR contacts with DQ1-bound peptides. For example, CDR3α F95 made 29 of a total of 36 TCR contacts to the UL15 peptide (20 of 30 to PMM peptide and 25 of 35 to MBP) ( Table 1 ). The side chain of CDR3α F95 bound in a pocket created by peptide P2, P3 and P5 side chains while the backbone of F95 formed a hydrogen bond with peptide P5 Lys/Arg. Crossreactivity by this self-reactive TCR is thus closely related to its tilted binding mode. We previously performed alanine-scanning mutagenesis of Hy.1B11 TCR residues that formed side chain interactions with the DQ1/MBP peptide complex (except those residues that were already alanine or glycine) [27] . Interestingly, the SPR-binding data for these mutants correlated well with computed ΔΔG values for an alanine scan of TCR residues contacting peptide or DQ1 (programme Robetta) ( Supplementary Table S5a ) [40] . Both approaches identified CDR3α E98 as the energetically most important TCR contact residue: in our SPR experiments the CDR3α E98A mutant showed little residual binding even at high TCR concentrations, and the Robetta programme assigned the highest ΔΔG values to this residue (9.72 for binding to DQ1/MBP). The SPR experiment also showed that the CDR3α F95A mutation greatly diminished peptide/DQ1 binding ( K d >250 μM), yet the effect of the CDR3α E98A mutant was even more severe. This result correlated well with the lower ΔΔG value (3.87) assigned to CDR3α F95 by the programme. This computational approach was then used to compare the three TCR–pMHC complexes, using separate alanine scans for DQ1 and peptide residues contacting TCR ( Supplementary Table S5b ). The results indicated that the CDR3α E98–DQ1α R61 interaction was substantially stronger than any other interaction among TCR, DQ1 and peptide, a result that correlated well with the SPR data. The data also suggested similar energetic contributions for the interaction of TCR CDR3α F95 with the three DQ1/peptide complexes, again in agreement with the experimental data. The experimental and computational data thus support the conclusion that these two residues of the TCR CDR3α loop dominate the energetic landscape of Hy.1B11 TCR binding to the three DQ1/peptide complexes. As both residues lie on the same CDR loop, conformational changes in this loop resulting in loss of binding contributions by F95 and/or E98 would be energetically highly unfavourable. The structure of unbound Hy.1B11 TCR is presently not available, and we therefore do not know whether the CDR3α loop is rigid or assumes similar conformations upon interaction with the three studied DQ1/peptide complexes. The highly crossreactive murine YAe62 TCR offers an interesting comparison to Hy.1B11 TCR. This TCR originated from mice in which negative selection was impaired due to covalent linkage of a single peptide into the MHCII binding groove (I-A b ) [41] . This TCR showed a high degree of peptide crossreactivity, MHC alloreactivity and even bound to a MHC class I/peptide complex [42] . Like Hy.1B11, YAe62 TCR bound in a tilted orientation to the MHCII/peptide surface, even though the tilt was not as severe as for Hy.1B11 (limited MHC contacts were made by the germline-encoded CDR1α and 2α loops of YAe62) [43] . YAe62 peptide contacts were severely limited and 69% of peptide contacts were made by a single aromatic residue located at the tip of the CDR3β loop (W95) ( Supplementary Fig. S5 ). This tryptophan residue bound in a pocket between the peptide and the I-A α1 helix, and it formed many contacts to P5 Lys as well as more limited contacts to P3 Lys and P6 Ala. Analogous to Hy.1B11 TCR, W95 also formed a main-chain hydrogen bond (to the MHC α1 helix) [43] . YAe62 was more crossreactive than Hy.1B11 because peptide specificity was largely limited to P5 Lys, whereas Hy.1B11 showed specificity for both P3 Phe and P5 Lys. Overall, the tilted-binding mode had similar consequences for engagement of MHCII and peptide: (1) TCR interactions with the MHCII β1 helix were greatly reduced; (2) a single aromatic residue located at the tip of a CDR3 loop formed most of the contacts with the peptide (CDR3α F95 for Hy.1B11, CDR3β W95 for YAe62); (3) one of the CDR3 loops formed few or no contacts with the peptide (CDR3β in Hy.1B11-DQ1/MBP, CDR3α in YAe62-IA b /3K). A tilted-binding mode can thus contribute to crossreactivity by focusing TCR specificity to a small part of the MHC-bound peptide. A tilted-binding mode was also identified for binding of the murine γδ TCR G8 to the MHC class Ib molecule T22. T22 does not bind a ligand and the C terminus of its α2 helix is unravelled, exposing the underlying β-sheet platform. The long TCR CDR3δ loop bound in this cavity and formed a large fraction of the interface with T22. In contrast, CDR1δ, CDR2δ and CDR3γ made small contributions to the binding interface [44] . While their interaction partners are very different (a MHC class Ib molecule without bound ligand versus a MHC class II–peptide complex), there are some similarities to Hy.1B11 TCR, in particular a tilted-binding mode and digit-type insertion of a single CDR3 loop into the groove. In several structures that have been reported, TCR crossreactivity involved major conformational changes of TCR loops, in particular the CDR3 loops [16] , [17] , [45] . In addition, conformational changes of bound peptides and less frequently conformational adjustments in the MHC molecule contributed to TCR crossreactivity [17] . For example, the alloreactive BM3.3 TCR showed major conformational changes in the CDR3α loop in TCR-pMHC structures involving two dissimilar peptides. In the structure with the high-affinity H-2K b /pBM1 peptide complex, the CDR3α loop was bent away from the peptide-binding groove. In contrast, CDR3α formed a substantial number of peptide contacts with the low-affinity H-2K b /VSV8 peptide complex. In addition, the BM3.3 TCR was shifted 1.2 Å towards the peptide C terminus and rotated by 5° in the structure involving the VSV8 peptide [16] . Alloreactivity can also occur without substantial conformational changes. The LC13 TCR recognized an EBV peptide bound to HLA-B*0801 and was alloreactive to HLA-B44 allotypes (B*4402 and B*4405) [46] . It bound with a similar orientation to HLA-B*0801/EBV and HLA-B*4405/ABCD3 peptide complexes, despite extensive MHC polymorphisms [46] . Hy.1B11 TCR did not show any domain movement or substantial adjustment of TCR CDR loops to accommodate differences in TCR-interacting peptide residues. We attribute this result to key interactions made by two residues at the tip of the CDR3α loop: the important interaction of CDR3α F95 with P2, P3 and P5 peptide residues, as well as the prominent energetic role of the CDR3α E98–DQ1α R61 interaction, which is part of a complex hydrogen bonding network. Ob.1A12 TCR showed similar interactions by the CDR3 loops with HLA-DR15-bound MBP and bacterial engA peptides, but there were significant differences in the conformation of the germline-encoded CDR2α and CDR2β loops [23] , [35] . No transgenic mouse model of Hy.1B11 TCR /HLA-DQ1 is available for testing the ability of PMM and UL15 peptides to induce CNS inflammation as had been performed for engA peptide in Ob.1A12 TCR/HLA-DR15 transgenic mice. Further, processing of PMM and UL15 peptides from complete microbial antigens was not tested. It is important to note that substantial changes in TCR and/or peptide conformation have been observed for sets of structures involving crossreactive peptides, despite sequence homology/identity among primary TCR contact residues. For example, the A6 TCR was specific for the Tax 11–19 peptide of the human retrovirus HTLV-1 and crossreacted with the Tel1p peptide from Saccharomyces cerevisiae . These two peptides shared sequence identity at four positions, including the primary TCR contacts P5 Tyr and P8 Tyr [47] . Nevertheless, there were substantial differences in the conformation of the peptide, the TCR and even the MHC molecule (HLA-A2) in trimolecular complexes involving Tax and Tel1p peptides [17] , [48] . In the structure with the Tel1p peptide, the P5 Tyr exhibited a 100° rotation around χ 1, resulting in a 9.6 Å displacement of the tyrosine hydroxyl. This conformational change was accompanied by a reorganization of the HLA-A2 α2 helix as well as a large distortion of the central pocket between the CDR3α and CDR3β loops (due to a 4.5 Å displacement of the apex of CDR3β) [17] . Comparison of the three Hy.1B11 TCR structures shows how a tilted TCR-binding mode focuses specificity to a short segment of the DQ1-bound peptide. These data thus provide a structural basis for crossreactivity by a self-reactive TCR from a patient with an autoimmune disease. Protein expression and complex formation Hy.1B11 TCR (TRAV13-1*02, TRAJ48*01, non-nucleotide encoded sequence: G ; TRBV7-3*01, TRBD2*01, TRBJ2-3*01, non-nucleotide encoded sequence: CCTCGGCCCT) was refolded from individual chains produced in E. coli [27] , [36] . Either the UL15 154–166 or PMM 260–274 peptide was attached to the N terminus of the TCRβ chain through a flexible octapeptide linker (GGSGGGGG), as reported by Hennecke and Wiley [49] . The chains were individually cloned into the pET22b vector and expressed as inclusion bodies in BL21(DE3) E. coli cells (Novagen). Purified inclusion bodies were solubilized in 6 M guanidine hydrochloride, 10 mM dithiothreitol and 10 mM EDTA. To initiate refolding, TCR α and β chains were diluted at a 1:1 molar ratio to a concentration of 25 μg ml −1 of each chain in a chilled refolding buffer containing 4.5 M urea, 0.55 M L -arginine-HCl, 100 mM Tris–HCl, pH 8.2, 1 mM GSH and 0.1 mM GSSH. The refolding mix was allowed to stand undisturbed for 40 h at 4 °C. After extensive dialysis (4 × ) in 10 mM Tris–HCl (pH 8.0), refolded TCR was concentrated to 1 mg ml −1 . The refolded protein was purified by anion-exchange chromatography using Poros PI (Applied Biosystems) followed by further purification using a MonoQ (GE Healthcare) column. DQ1 was produced in glycosylation-deficient Lec3.2.8.1 cells. The CLIP peptide was attached to the N terminus of the DQ1β chain using a linker with a thrombin cleavage site, and the two chains were cloned into a vector that drove expression of glutamine synthetase for selection of transfected clones in glutamine-deficient media. Stable clones were produced under methionine sulphoximine selection and tested for DQ1 secretion by western blotting. The clone with the highest DQ1 production level was expanded in a hollow fibre bioreactor (Acusyst MiniMax, Biovest International) and secreted DQ1 was affinity-purified using mAb 9.3.F10 (ATCC, Manassas, VA, USA). C-terminal Fos and Jun leucine zipper dimerization domains were used to facilitate DQ1 heterodimer formation and later removed by V8 protease cleavage [27] . Following cleavage of the CLIP peptide linker, complexes were formed by permitting binding of TCRβ chain-linked UL15 154–166 or PMM 260–274 peptide to the DQ1-binding site. TCR, DQ1 and HLA-DM were incubated at a molar ratio of 6:4:1 for 18 h at 25 °C at a pH of 5.4, and the complex was separated from components by gel filtration (Superdex S200 column, GE Healthcare) and anion-exchange chromatography (MonoQ, GE Healthcare). Crystallization and data collection The protein complexes were determined to be pure and monodisperse by SDS–PAGE and isoelectric focusing PAGE. TCR–pMHC complexes were concentrated to 7 mg ml −1 in 5 mM HEPES (pH 7.4). Crystals used for data collection (both complexes) were grown using the hanging-drop vapor-diffusion method against a reservoir of 0.1 M ammonium sulphate, 8–11% PEG 8000 and 50 mM sodium citrate (pH 6.1) at 23 °C. These crystallization conditions were very similar to those for the Hy.1B11-MBP/DQ1 complex. Crystals were cryoprotected by addition of ethylene glycol to 25%. Data were collected at 100 K at the Advanced Photon Source, Argonne National Laboratories at beamlines 24-IDE (Hy.1B11-DQ1/PMM) and 24-IDC (Hy.1B11-DQ1/UL15). The data were processed with HKL2000 (ref. 50 ). Structure determination and refinement Structures were determined by molecular replacement using PHASER software [51] . Hy.1B11 TCR and HLA-DQ1 without the peptide from PDB entry 3PL6 were used for molecular replacement. PHASER gave a clear and unambiguous solution that could be reproduced using the MOLREP programme [51] , [52] . Initial stages of refinement and rebuilding were carried out using crystallography and nuclear magnetic resonance system (CNS) and COOT [53] , [54] . Later stages of refinement were completed using PHENIX [55] . Structures were refined through several rounds of manual rebuilding interspersed with positional and temperature factor refinement. Stereochemical parameters were evaluated with PROCHECK and found to be within reasonable limits [56] . Buried surface area calculations were performed using AREAIMOL using a probe radius of 1.4 Å (ref. 57 ). All figures were made using PYMOL ( http://www.pymol.org/ ). Atomic contacts were determined using CONTACT as implemented in the CCP4i (CCP4 suite) [58] ; atoms within a 4 Å distance of each other were considered to be in contact. SPR experiments The interaction of Hy.1B11 TCR with DQ1/MBP, DQ1/UL15 or DQ1/PMM was assessed by surface plasmon resonance using a BIAcore 3000 instrument (GE Healthcare). In each case, DQ1 loaded with the appropriate peptide was captured on a BIAcore streptavidin chip through a biotinylated C-terminal BirA tag. After immobilization of DQ1/peptide complexes (~1,500 resonance units, RU), soluble monomeric WT or mutant Hy.1B11 TCR was injected at a range of different concentrations. A flow cell with immobilized DQ1/CLIP was used to assess background binding. For the measurements at 37 °C, the TCR Hy.1B11 was immobilized using its biotinylated C-terminal BirA tag on the streptavidin surface (1,500 or 2,000 RU) using TCR Ob.1A12 as control and pMHC complexes at various concentrations were injected. All measurements were minimally performed in duplicate. BIAevaluation software version 4.1 was used for data analysis. Equilibrium K d values were obtained by nonlinear curve fitting of background-subtracted data using steady state affinity fitting in BIAevaluation version 4.1. Error estimates were propagated from the SE of the K A . Peptide-binding experiments A competition assay involving a biotinylated MBP 85-99 peptide was used to assess the binding of a panel of unlabelled MBP analogues with substitutions at DQ1 anchor positions (P1, P4, P6 and P9). DQ1/CLIP (100 nM) was incubated overnight at room temperature in citrate buffer (pH 5.2) with biotinylated MBP 85–99 (400 nM), HLA-DM (30 nM) and MBP analogue peptides (30, 10, 3, 1 and 0.3 μM). DQ1/peptide complexes were then captured on an ELISA plate using mAb 9.3.F10 (0.4 μg per well). Following four washes with Tris-buffered saline, 0.05% Tween 20 (TBST), nonspecific binding sites were blocked using DELFIA assay buffer (Perkin Elmer) (2 h, RT, followed by several washes). An aliquot of each peptide-binding reaction (50 μl) and of assay buffer (75 μl) were added to each well (1 h at RT, followed by four washes). Europium-labeled streptavidin (100 μl, diluted 1:2,000 in DELFIA assay buffer) was added to each well (1 h incubation, followed by six washes). DELFIA enhancement solution (100 μl, Perkin Elmer) was then added and europium fluorescence was quantified after a 30 min incubation using a Victor [3] plate reader (Perkin Elmer). T cell assay Proliferation assays with the Hy.1B11 T cell clone were performed using EBV-transformed B-cell line 9009 ( DQA1 *0102, DQB1 *0502) as antigen-presenting cells. B cells were irradiated (5,000 rads) and treated with 50 μg ml −1 mitomycin C (Calbiochem) for 30 min at 37 °C. Assays were set up in 96-well U bottom plates with 5 × 10 4 T cells and 10 4 B cells in 0.2 ml of serum-free AIM-V media supplemented with 2 mM Glutamax. Peptides were tested in triplicates at concentrations ranging from 50 nM to 50 μM. After 72 h of co-culture, T cell proliferation was determined by [ 3 H]-thymidine incorporation. Accession codes: The structures have been deposited in the PDB with accession codes 4GRL (Hy.1B11-DQ1/PMM) and 4MAY (Hy.1B11-DQ1/UL15) How to cite this article: Sethi, D. K. et al . Crossreactivity of a human autoimmune TCR is dominated by a single TCR Loop. Nat. Commun. 4:2623 doi: 10.1038/ncomms3623 (2013).